Macrophage-inducible C-type lectin underlies obesity-induced adipose tissue fibrosis In obesity, a paracrine loop between adipocytes and macrophages augments chronic inflammation of adipose tissue, thereby inducing systemic insulin resistance and ectopic lipid accumulation. Obese adipose tissue contains a unique histological structure termed crown-like structure (CLS), where adipocyte-macrophage crosstalk is known to occur in close proximity. Here we show that Macrophage-inducible C-type lectin (Mincle), a pathogen sensor for Mycobacterium tuberculosis , is localized to macrophages in CLS, the number of which correlates with the extent of interstitial fibrosis. Mincle induces obesity-induced adipose tissue fibrosis, thereby leading to steatosis and insulin resistance in liver. We further show that Mincle in macrophages is crucial for CLS formation, expression of fibrosis-related genes and myofibroblast activation. This study indicates that Mincle, when activated by an endogenous ligand released from dying adipocytes, is involved in adipose tissue remodelling, thereby suggesting that sustained interactions between adipocytes and macrophages within CLS could be a therapeutic target for obesity-induced ectopic lipid accumulation. Obesity is a state of chronic, low-grade inflammation [1] , [2] . Indeed, adipose tissue in obesity is characterized by adipocyte hypertrophy, followed by increased angiogenesis, immune cell infiltration, extracellular matrix overproduction, which is referred to as ‘adipose tissue remodelling’ [3] , [4] . As a molecular mechanism, we have provided evidence that a paracrine loop involving saturated fatty acids and tumour necrosis factor-α (TNFα) derived from adipocytes and macrophages, respectively, establishes a vicious cycle, thereby accelerating the inflammatory change in obese adipose tissue [5] . It is conceivable that increased adipose tissue inflammation stimulates adipocyte lipolysis and tissue fibrosis, and thus enhances the release of free fatty acids from the adipose tissue, which may be accumulated in non-adipose tissue such as liver and skeletal muscle, as ectopic fat, and induce a variety of metabolic abnormalities called lipotoxicity [3] , [4] . In this regard, Khan et al . [6] reported that mice lacking collagen VI, which is expressed abundantly in adipose tissue, exhibit the uninhibited adipose tissue expansion and substantial improvement in insulin sensitivity on a high-fat diet (HFD). Although recent evidence suggests a role for obesity-induced hypoxic state [7] , [8] , the molecular mechanisms underlying adipose tissue fibrosis are still largely unknown. As the site of crosstalk between adipocytes and macrophages, there is a unique structure in obese adipose tissue called crown-like structure (CLS), where macrophages are considered to scavenge the residual lipid droplets of dead adipocytes [9] , [10] . Histologically, proinflammatory M1 macrophages aggregate to constitute CLS in obese adipose tissue of humans and rodents. On the other hand, M2 macrophages are scattered in the interstitial spaces between adipocytes [10] . Notably, the number of CLS is positively correlated with systemic insulin resistance in obese subjects [11] , [12] , suggesting the pathophysiologic role of CLS in adipose tissue inflammation and systemic energy metabolism. However, how CLS is formed in adipose tissue during the course of obesity and how it is involved in adipose tissue remodelling are poorly understood. Macrophage-inducible C-type lectin (Mincle, Clec4e or Clecsf9) is a pathogen sensor that recognizes pathogenic fungi and Mycobacterium tuberculosis [13] , [14] , [15] , [16] , and as the name implies, it is induced in macrophages by lipopolysaccharide through Toll-like receptor 4 (TLR4; ref. 17 ). We previously reported that saturated fatty acids also induce Mincle expression in macrophages through TLR4 (ref. 18 ). Moreover, the obesity-induced increase in Mincle expression in adipose tissue is markedly attenuated in C3H/HeJ mice with defective TLR4 signalling relative to control C3H/HeN mice [18] . Yamasaki et al . reported that Mincle can sense cell death as well to induce proinflammatory cytokine production and suggested the role of Mincle in sterile inflammation [19] . We have recently demonstrated that Mincle is induced in adipose tissue macrophages during the interaction between adipocytes and macrophages, at least partly, through the saturated fatty acid/TLR4/NF-κB pathway [18] . It is currently unclear whether Mincle regulates adipose tissue inflammation and thus systemic energy metabolism in obesity, and if so, how it does remains to be elucidated. Here we show that Mincle , when induced during the development of obesity, is localized to macrophages constituting CLS in adipose tissue. Interestingly, Mincle KO mice are protected against obesity-induced CLS formation and adipose tissue fibrosis, followed by reduced ectopic lipid accumulation and insulin resistance in the liver. On the other hand, treatment with trehalose-6,6′-dimycolate (TDM), a mycobacterial cell wall glycolipid that is known to be a Mincle ligand [13] , induces CLS formation and interstitial fibrosis in adipose tissue in mice. Mincle stimulation also induces potently expression of fibrosis-related genes in macrophages in vitro . This study provides evidence that Mincle has a role in the crosstalk between adipocytes and macrophages in CLS, thereby leading to activation of fibrogenic programme. Our data also suggest that antagonism of Mincle in macrophages offers a novel therapeutic strategy to prevent or treat obesity-induced adipose tissue fibrosis and thus ectopic lipid accumulation. Adipose tissue Mincle expression in obesity We previously reported that Mincle expression is markedly upregulated in adipose tissue macrophages in obesity [18] . In this study, we first examined the time course of Mincle mRNA expression in epididymal fat tissue of wild-type mice fed a HFD and found that Mincle mRNA expression was roughly constant in wild-type mice fed a standard diet (SD) throughout the experimental period. On the other hand, Mincle mRNA expression was significantly increased in wild-type mice fed a HFD relative to those fed a SD at 16 weeks and gradually increased up to 50 weeks. There was no significant difference in expression of Emr1 , which encodes macrophage marker F4/80, between 16 and 50 weeks ( Fig. 1a ). Mincle mRNA expression was also increased in liver to a lesser extent than epididymal fat tissue ( Fig. 1b ). At 16 weeks, Mincle mRNA expression was markedly high in epididymal fat tissue relative to subcutaneous fat tissue, which was roughly in parallel with Emr1 mRNA expression ( Fig. 1c ). In the stromal-vascular fraction (SVF) from epididymal fat tissue of genetically obese ob/ob mice, Mincle mRNA was exclusively expressed in CD45 + CD11b + F4/80 + cells or macrophages ( Fig. 1d ). In line with this, flow cytometric analysis revealed that obesity markedly increased the number of Mincle-positive macrophages, whereas there was no appreciable Mincle expression in other immune cells ( Fig. 1e ). 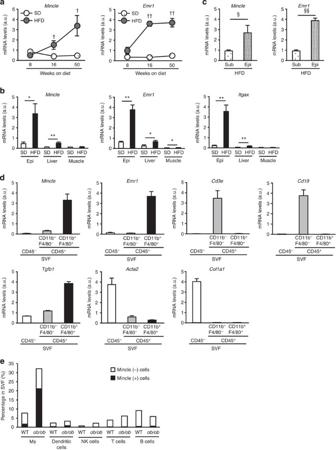Figure 1: Adipose tissueMincleexpression and Mincle-expressing cells in obese adipose tissue. (a) Time course ofMinclemRNA andEmr1(F4/80) expression in epididymal fat tissue of wild-type mice fed a HFD or a SD for up to 50 weeks. Values are mean±s.e.m. The data are analysed by unpairedt-test;n=5 to 11;†P<0.05,††P<0.01 versus SD at each time point. (b) mRNA expression ofMincle,Emr1andItgax(CD11c) in epididymal fat tissue (Epi), liver and skeletal muscle in wild-type mice fed a HFD for 50 weeks. Values are mean±s.e.m. The data are analysed by unpairedt-test;n=5 to 10;*P<0.05,**P<0.01. (c)MinclemRNA expression in epididymal (Epi) and subcutaneous (Sub) fat tissues of wild-type mice on a HFD for 16 weeks. Values are mean±s.e.m. The data are analysed by unpairedt-test;n=11;§P<0.05,§§P<0.01. (d) mRNA expression ofMincle,Emr1, Acta2(αSMA), and other cell type markers in CD45−, CD45+CD11b−F4/80−and CD45+CD11b+F4/80+cells isolated from SVF. Values are mean±s.e.m.;n=4. (e) Percentage of Mincle-expressing cells in various immune cells in SVF. Values are the average of four samples. Figure 1: Adipose tissue Mincle expression and Mincle-expressing cells in obese adipose tissue. ( a ) Time course of Mincle mRNA and Emr1 (F4/80) expression in epididymal fat tissue of wild-type mice fed a HFD or a SD for up to 50 weeks. Values are mean±s.e.m. The data are analysed by unpaired t -test; n =5 to 11; † P <0.05, †† P <0.01 versus SD at each time point. ( b ) mRNA expression of Mincle , Emr1 and Itgax (CD11c) in epididymal fat tissue (Epi), liver and skeletal muscle in wild-type mice fed a HFD for 50 weeks. Values are mean±s.e.m. The data are analysed by unpaired t -test; n =5 to 10; *P <0.05, **P <0.01. ( c ) Mincle mRNA expression in epididymal (Epi) and subcutaneous (Sub) fat tissues of wild-type mice on a HFD for 16 weeks. Values are mean±s.e.m. The data are analysed by unpaired t -test; n =11; § P <0.05, §§ P <0.01. ( d ) mRNA expression of Mincle , Emr1, Acta2 (αSMA), and other cell type markers in CD45 − , CD45 + CD11b − F4/80 − and CD45 + CD11b + F4/80 + cells isolated from SVF. Values are mean±s.e.m. ; n =4. ( e ) Percentage of Mincle-expressing cells in various immune cells in SVF. Values are the average of four samples. Full size image Altered lipid distribution in Mincle KO mice We next examined the metabolic phenotypes of Mincle KO mice at 16 weeks of HFD feeding. There was no appreciable difference in body weight and subcutaneous fat weight between the genotypes ( Fig. 2a and Supplementary Fig. 1a ). The epididymal fat weight was significantly increased with reciprocal reduction of the liver weight in Mincle KO mice relative to wild-type mice on a HFD ( Fig. 2a and Supplementary Fig. 1a ). Histological examination revealed that hepatic steatosis was markedly attenuated in Mincle KO mice relative to wild-type mice ( Fig. 2b ). Consistently, hepatic triglyceride content and serum free fatty acid (FFA) and alanine aminotransferase (ALT) concentrations were significantly reduced in Mincle KO mice relative to wild-type mice ( Fig. 2c,d ). Basically, similar results were obtained in Mincle KO mice fed a HFD for 50 weeks ( Supplementary Fig. 2a,b ). On the other hand, at 8 weeks of HFD feeding when there was no apparent difference in Mincle expression in epididymal fat tissue between the diets ( Fig. 1a ), we did not observe any difference in the body weight and tissue weights between the genotypes ( Supplementary Fig. 3 ). These observations suggest the altered lipid distribution in adipose tissue and liver in Mincle KO mice on a HFD. 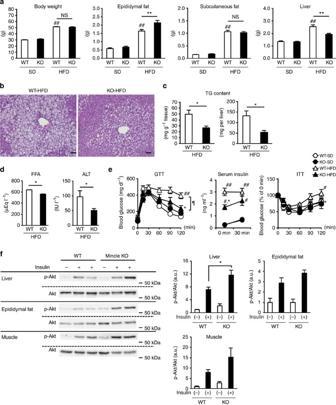Figure 2: Altered lipid distribution between adipose tissue and liver inMincleKO mice. (a) Body weight and fat and liver weights ofMincleKO and wild-type mice at 16 weeks. Values are mean±s.e.m. The data are analysed by analysis of variance (ANOVA) followed by Tukey–Kramer test.##P<0.01 versus WT-SD, **P<0.01. NS, not significant;n=11 to 13. (b–d) Representative hematoxylin and eosin staining of the liver (b), hepatic triglyceride (TG) content (c) and serum FFA and ALT concentrations (d) inMincleKO and wild-type mice at 16 weeks. Original magnification, × 200; Scale bar, 50 μm. Values are mean±s.e.m. The data are analysed by unpairedt-test. *P<0.05;n=11 to 13. (e,f) Glucose metabolism inMincleKO and wild-type mice fed a HFD for 50 weeks;n=5 to 8. (e) Glucose and insulin tolerance tests. Values are mean±s.e.m. The data are analysed by ANOVA followed by Tukey–Kramer test.#P<0.05,##P<0.01 versus WT-SD and *P<0.05 versus WT-HFD at each point.¶P<0.05 assessed by ANOVA with repeated-measures analysis. (f) Western blotting of phosphorylated Akt (Thr308) in liver, epididymal fat tissue and soleus muscle. Values are mean±s.e.m. The data are analyzed by ANOVA followed by Tukey–Kramer test; *P<0.05. Figure 2: Altered lipid distribution between adipose tissue and liver in Mincle KO mice. ( a ) Body weight and fat and liver weights of Mincle KO and wild-type mice at 16 weeks. Values are mean±s.e.m. The data are analysed by analysis of variance (ANOVA) followed by Tukey–Kramer test. ## P <0.01 versus WT-SD, ** P <0.01. NS, not significant; n =11 to 13. ( b – d ) Representative hematoxylin and eosin staining of the liver ( b ), hepatic triglyceride (TG) content ( c ) and serum FFA and ALT concentrations ( d ) in Mincle KO and wild-type mice at 16 weeks. Original magnification, × 200; Scale bar, 50 μm. Values are mean±s.e.m. The data are analysed by unpaired t -test. * P <0.05; n =11 to 13. ( e , f ) Glucose metabolism in Mincle KO and wild-type mice fed a HFD for 50 weeks; n =5 to 8. ( e ) Glucose and insulin tolerance tests. Values are mean±s.e.m. The data are analysed by ANOVA followed by Tukey–Kramer test. # P <0.05, ## P <0.01 versus WT-SD and * P <0.05 versus WT-HFD at each point. ¶ P <0.05 assessed by ANOVA with repeated-measures analysis. ( f ) Western blotting of phosphorylated Akt (Thr308) in liver, epididymal fat tissue and soleus muscle. Values are mean±s.e.m. The data are analyzed by ANOVA followed by Tukey–Kramer test; * P <0.05. Full size image Ameliorated glucose metabolism in Mincle KO mice We performed the glucose tolerance test at 16 weeks of HFD feeding and found that Mincle KO mice showed better glucose tolerance and lower serum insulin concentrations than wild-type mice ( Supplementary Fig. 1b ). Moreover, the insulin-induced phosphorylation of Akt was significantly increased in the liver of Mincle KO mice relative to that of wild-type mice ( Supplementary Fig. 1c ). The phosphorylated Akt levels also tended to increase in the adipose tissue and skeletal muscle in Mincle KO mice, which did not reach statistical significance. In addition, there was a slight decrease in the insulin-positive area and the number of Ki67-positive cells in the pancreas of Mincle KO mice relative to that of wild-type mice, whereas the islet area and glucagon-positive area did not differ between the genotypes ( Supplementary Fig. 4 ). These observations suggest that reduced insulin resistance in the liver leads to better glucose tolerance in Mincle KO mice. We confirmed similar results at 50 weeks ( Fig. 2e,f and Supplementary Fig. 2c ). Collectively, HFD-induced insulin resistance was ameliorated in the liver of Mincle KO mice along with reduced hepatic lipid accumulation. Reduced adipose tissue fibrosis in Mincle KO mice Histological analysis of epididymal fat tissue revealed that adipocyte cell size appears to be increased in Mincle KO mice relative to wild-type mice on a HFD for 16 weeks, whereas there was no significant difference in the number of adipocytes ( Fig. 3a ). In this study, mRNA expression of genes related to adipogenesis, lipogenesis, lipolysis and β-oxidation did not differ between the genotypes ( Supplementary Fig. 5 ). In addition, flow cytometric analysis showed no significant difference in the ratio of each immune cell to the SVF ( Supplementary Fig. 6 ). On the other hand, Masson’s trichrome staining revealed extensive interstitial fibrosis in epididymal fat tissue of wild-type mice, which is markedly suppressed in Mincle KO mice ( Fig. 3b,c ). We also obtained similar results by Sirius red staining and measurement of total collagen content ( Fig. 3d–f ). Consistently, there was a significant decrease in the area of αSMA-positive cells or myofibroblasts in Mincle KO mice relative to wild-type mice ( Fig. 3g,h ). Interestingly, there was no significant difference in total collagen content of subcutaneous fat tissue between the genotypes ( Fig. 3f ). We confirmed these results in Mincle KO mice fed a HFD for 50 weeks ( Supplementary Fig. 2d,e ). Collectively, these observations indicate reduced interstitial fibrosis in epididymal fat tissue of Mincle KO mice relative to wild-type mice. 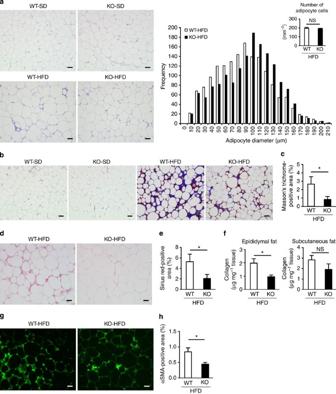Figure 3: Reduced interstitial fibrosis in adipose tissue ofMincleKO mice. MincleKO and wild-type mice were fed a HFD or a SD for 16 weeks. (a) Representative hematoxylin and eosin staining, the histogram of adipocyte diameters in epididymal fat tissue. Inset, the number of adipocyte cells in epididymal fat tissue. (b,c) Representative Masson’s trichrome staining (b) and quantification of Masson’s trichrome-positive area (identical with interstitial fibrosis) (c) in epididymal fat tissue. (d,e) Representative Sirius red staining (d) and quantification of Sirius red-positive area (e) in epididymal fat tissue. (f) Total collagen contents in epididymal and subcutaneous fat tissues. (g,h) Representative αSMA staining (g) and quantification of αSMA-positive area (h) in epididymal fat tissue. Original magnification, × 200; Scale bar, 50 μm. Values are mean±s.e.m. The data are analysed by unpairedt-test. *P<0.05; NS, not significant;n=11 to 13. Figure 3: Reduced interstitial fibrosis in adipose tissue of Mincle KO mice. Mincle KO and wild-type mice were fed a HFD or a SD for 16 weeks. ( a ) Representative hematoxylin and eosin staining, the histogram of adipocyte diameters in epididymal fat tissue. Inset, the number of adipocyte cells in epididymal fat tissue. ( b , c ) Representative Masson’s trichrome staining ( b ) and quantification of Masson’s trichrome-positive area (identical with interstitial fibrosis) ( c ) in epididymal fat tissue. ( d , e ) Representative Sirius red staining ( d ) and quantification of Sirius red-positive area ( e ) in epididymal fat tissue. ( f ) Total collagen contents in epididymal and subcutaneous fat tissues. ( g , h ) Representative αSMA staining ( g ) and quantification of αSMA-positive area ( h ) in epididymal fat tissue. Original magnification, × 200; Scale bar, 50 μm. Values are mean±s.e.m. The data are analysed by unpaired t -test. * P <0.05; NS, not significant; n =11 to 13. Full size image Since Mincle is expressed selectively in adipose tissue macrophages ( Fig. 1e ), we next performed bone marrow transplantation (BMT) experiments to confirm the role of Mincle in bone marrow-derived cells. In this study, the substitution rate of BMT was more than 90% ( Supplementary Fig. 7a ). Mincle mRNA expression in epididymal fat tissue was almost negligible in bone marrow-specific Mincle KO mice (Mincle KO-BM mice) compared with the control mice (EGFP-BM mice) ( Supplementary Fig. 7b ), suggesting the macrophage-selective expression of Mincle ( Fig. 1d ). Under these experimental conditions, we confirmed that Mincle deficiency protected against HFD-induced adipose tissue fibrosis ( Supplementary Fig. 7c ). Reduced CLS formation in adipose tissue of Mincle KO mice To determine the localization of Mincle expression in obese adipose tissue, we performed in situ hybridization analysis and found that Mincle occurs in some of the macrophages constituting CLS in epididymal fat tissue ( Fig. 4a,b ). Flow cytometric analysis revealed that CD11b + F4/80 lo cells isolated from the SVF showed higher Mincle mRNA expression than CD11b + F4/80 hi cells ( Fig. 4c ). CD11b + F4/80 lo cells expressed higher Itgax (CD11c) and lower Mrc1 (CD206) mRNA levels than CD11b + F4/80 hi cells. These observations are consistent with our previous data that Mincle is expressed selectively in proinflammatory M1 macrophages in vitro [18] . Interestingly, the CLS density in Mincle KO mice was markedly reduced relative to wild-type mice ( Fig. 4d,e ). Moreover, there was a significant decrease in Tnfa (TNFα) mRNA expression in Mincle KO mice relative to wild-type mice on a HFD ( Fig. 4f ). On the other hand, there was no significant difference in macrophage number ( Fig. 4e ) and polarization ( Fig. 4f and Supplementary Fig. 6b ) between the genotypes. By double-immunofluorescent staining of F4/80 (green) and collagen I (red), we observed the adjacent spatial relationship between CLS and fibrotic regions ( Fig. 4g ). The CLS density was positively correlated with the extent of adipose tissue fibrosis determined by Masson’s trichrome and Sirius red stainings ( Fig. 4h ). Collectively, these observations suggest that Mincle-mediated CLS formation has a role in interstitial fibrosis in adipose tissue. 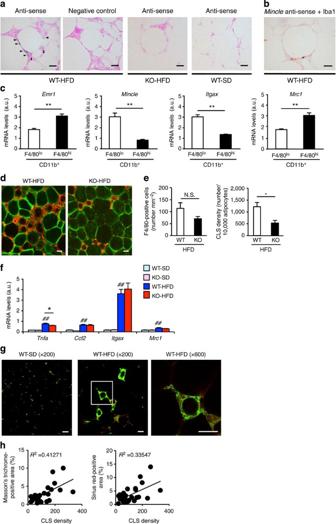Figure 4: Reduced CLS formation in adipose tissue ofMincleKO mice. (a) Representativein situhybridization forMinclemRNA in epididymal fat tissue of wild-type andMincleKO mice fed a HFD for 16 weeks. The sections were hybridized with an anti-sense or a sense probe. (b) Double staining forMincle(blue) and Iba1, a macrophage marker (brown). Afterin situhybridization forMinclemRNA, the sections were immunostained with an anti-Iba1 antibody. Original magnification, × 400; Scale bars, 25 μm. (c) mRNA expression ofMincle,Emr1,ItgaxandMrc1(CD206) in CD11b+F4/80loand CD11b+F4/80hicells isolated from SVF. Values are mean±s.e.m. The data are analysed by unpairedt-test;n=4,**P<0.01. (d,e) Representative immunofluorescent staining of F4/80 (red) and perilipin (green) (d) and the number of F4/80-positive cells and crown-like structure (CLS) density (e) in epididymal fat tissue ofMincleKO and wild-type mice fed a HFD for 16 weeks. Original magnification, × 200; Scale bars, 50 μm. Values are mean±s.e.m. The data are analysed by unpairedt-test;n=6 to 8,*P<0.05. NS, not significant. (f) mRNA expression ofTnfa(TNFα),Ccl2(MCP-1),ItgaxandMrc1in epididymal fat tissue ofMincleKO and wild-type mice fed a HFD for 16 weeks. Values are mean±s.e.m. The data are analysed by ANOVA followed by Tukey–Kramer test.n=5 to 11.##P<0.01 versus WT-SD, *P<0.05. (g) Representative immunofluorescent staining of F4/80 (green) and collagen I (red) in epididymal fat tissue of wild-type mice fed a SD or a HFD for 16 weeks. Scale bar, 50 μm. (h) Linear regression analysis of correlations between Masson’s trichrome- or Sirius red-positive area and CLS density in epididymal fat tissue of wild-type mice fed a HFD for 16 to 20 weeks;n=24. Figure 4: Reduced CLS formation in adipose tissue of Mincle KO mice. ( a ) Representative in situ hybridization for Mincle mRNA in epididymal fat tissue of wild-type and Mincle KO mice fed a HFD for 16 weeks. The sections were hybridized with an anti-sense or a sense probe. ( b ) Double staining for Mincle (blue) and Iba1, a macrophage marker (brown). After in situ hybridization for Mincle mRNA, the sections were immunostained with an anti-Iba1 antibody. Original magnification, × 400; Scale bars, 25 μm. ( c ) mRNA expression of Mincle , Emr1 , Itgax and Mrc1 (CD206) in CD11b + F4/80 lo and CD11b + F4/80 hi cells isolated from SVF. Values are mean±s.e.m. The data are analysed by unpaired t -test; n =4, **P <0.01. ( d , e ) Representative immunofluorescent staining of F4/80 (red) and perilipin (green) ( d ) and the number of F4/80-positive cells and crown-like structure (CLS) density ( e ) in epididymal fat tissue of Mincle KO and wild-type mice fed a HFD for 16 weeks. Original magnification, × 200; Scale bars, 50 μm. Values are mean±s.e.m. The data are analysed by unpaired t -test; n =6 to 8, *P <0.05. NS, not significant. ( f ) mRNA expression of Tnfa (TNFα), Ccl2 (MCP-1), Itgax and Mrc1 in epididymal fat tissue of Mincle KO and wild-type mice fed a HFD for 16 weeks. Values are mean±s.e.m. The data are analysed by ANOVA followed by Tukey–Kramer test. n =5 to 11. ## P <0.01 versus WT-SD, * P <0.05. ( g ) Representative immunofluorescent staining of F4/80 (green) and collagen I (red) in epididymal fat tissue of wild-type mice fed a SD or a HFD for 16 weeks. Scale bar, 50 μm. ( h ) Linear regression analysis of correlations between Masson’s trichrome- or Sirius red-positive area and CLS density in epididymal fat tissue of wild-type mice fed a HFD for 16 to 20 weeks; n =24. Full size image Mincle-stimulated fibrogenic gene expression in macrophages To elucidate how Mincle regulates adipose tissue fibrosis, we performed DNA microarray analysis of peritoneal macrophages stimulated with TDM ( Fig. 5a ). A total of 179 genes were upregulated by TDM in wild-type macrophages and the effect was totally abolished in Mincle KO macrophages ( Supplementary Table 1 ), indicating the Mincle-specific activation by TDM. In addition to known chemokine and cytokine genes, pathway analysis using Reactome database ( http://www.reactome.org/ ) identified several large clusters related to tissue remodelling ( Supplementary Fig. 8 ). By quantitative real-time PCR, we confirmed that TDM treatment markedly increases mRNA expression of Tgfb1 (TGFβ1), Pdgfb and Timp1 ( Fig. 5b ), which regulate extracellular matrix (ECM) production, fibroblast proliferation and ECM degradation, respectively [20] . Since the Fc receptor common γ-chain (FcRγ)-spleen tyrosine kinase (Syk) cascade is shown to be downstream of Mincle signalling [19] , we examined the involvement of Syk in the induction of fibrosis-related genes. Treatment with a Syk-inhibitor suppressed dose-dependently the mRNA expression of Tgfb1 , Pdgfb and Timp1 along with Cxcl2 (MIP-2), a chemokine that is induced by the Mincle-Syk pathway [19] ( Fig. 5c ). These observations suggest that Mincle activation potently induces fibrosis-related genes through Syk in macrophages. 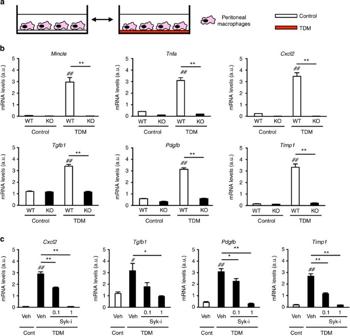Figure 5: Mincle-stimulated expression of fibrosis-related genes in macrophages. (a) Illustration of the TDM-stimulated experiments using peritoneal macrophages. (b) Effect of TDM stimulation for 24 h on mRNA expression ofMincle, inflammatory cytokines (TnfaandCxcl2(MIP-2)) and fibrosis-related genes (Tgfb1(TGFβ1),PdgfbandTimp1) in peritoneal macrophages fromMincleKO and wild-type mice. (c) Effect of Syk-inhibitor BAY61-3606 (0.1, 1 μM) on mRNA expression in wild-type peritoneal macrophages stimulated with TDM. Cont, Control; Syk-i, Syk-inhibitor; TDM, trehalose-6,6′-dimycolate; Veh, Vehicle. Values are mean±s.e.m. The data are analysed by ANOVA followed by Tukey–Kramer test;n=4,#P<0.05,##P<0.01 versus WT–Control or Veh–Control, *P<0.05, **P<0.01. Figure 5: Mincle-stimulated expression of fibrosis-related genes in macrophages. ( a ) Illustration of the TDM-stimulated experiments using peritoneal macrophages. ( b ) Effect of TDM stimulation for 24 h on mRNA expression of Mincle , inflammatory cytokines ( Tnfa and Cxcl2 (MIP-2)) and fibrosis-related genes ( Tgfb1 (TGFβ1), Pdgfb and Timp1 ) in peritoneal macrophages from Mincle KO and wild-type mice. ( c ) Effect of Syk-inhibitor BAY61-3606 (0.1, 1 μM) on mRNA expression in wild-type peritoneal macrophages stimulated with TDM. Cont, Control; Syk-i, Syk-inhibitor; TDM, trehalose-6,6′-dimycolate; Veh, Vehicle. Values are mean±s.e.m. The data are analysed by ANOVA followed by Tukey–Kramer test; n =4, # P <0.05, ## P <0.01 versus WT–Control or Veh–Control, * P <0.05, ** P <0.01. Full size image Mincle-stimulated increase of myofibroblasts in SVF Since activated fibroblasts or myofibroblasts are crucial for fibrogenesis in various tissues and organs [20] , [21] , we next examined the effect of Mincle stimulation of SVF that contains a variety of cell types such as immune cells, vascular cells and fibroblasts ( Fig. 6a ). The SVF was prepared from epididymal fat tissue of 9-week-old ob/ob mice; they showed high macrophage infiltration and Mincle expression relative to wild-type mice as reported [18] . Stimulation with TDM for 1 day significantly increased Mincle , Tnfa , Pdgfb and Timp1 mRNA expression in the SVF ( Fig. 6b ). The effect of Mincle stimulation was also observed after 3 days ( Fig. 6b ). Interestingly, mRNA expression of Acta2 , which encodes the myofibroblast marker αSMA, was significantly increased by Mincle stimulation ( Fig. 6b ). To address the effect of Mincle activation in macrophages on adipose tissue fibroblasts, we co-cultured peritoneal macrophages with CD45 − CD31 − cells prepared from the SVF of ob/ob mice which should abundantly include fibroblasts ( Fig. 6c ). Stimulation of the co-culture with TDM time-dependently increased mRNA expression of Acta2 , which was followed by the increase of Col1a1 (collagen I) mRNA expression ( Fig. 6d ). These observations strongly suggest that Mincle activation in macrophages effectively increases the number of myofibroblasts in adipose tissue. 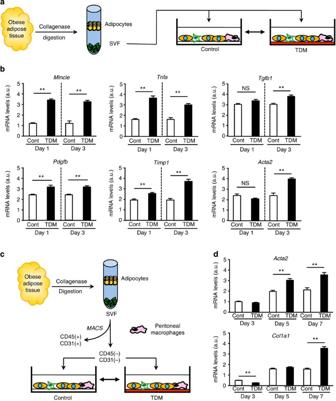Figure 6: Mincle-stimulated increase of myofibroblasts in SVF. (a) Illustration of the TDM-stimulated experiments using SVF. SVF prepared from epididymal fat tissue ofob/obmice was stimulated with TDM for up to 3 days. (b) Effect of TDM stimulation on mRNA expression ofMincle,Tnfa, fibrosis-related genes (Tgfb1,Pdgfb,Timp1) andActa2. Values are mean±s.e.m. The data are analysed by unpairedt-test;n=4, **P<0.01, NS, not significant. (c,d) Co-culture experiments of peritoneal macrophages and adipose tissue fibroblasts. (c) Illustration of the co-culture experiments using peritoneal macrophages and CD45−CD31−cells in SVF, rich in fibroblasts, prepared from epididymal fat tissue ofob/obmice using the magnetic cell sorting system (MACS). The cells were stimulated with TDM for up to 7 days. (d) Effect of TDM stimulation on mRNA expression ofActa2andCol1a1(collagen I). Values are mean±s.e.m. The data are analysed by unpairedt-test;n=4, **P<0.01. Figure 6: Mincle-stimulated increase of myofibroblasts in SVF. ( a ) Illustration of the TDM-stimulated experiments using SVF. SVF prepared from epididymal fat tissue of ob/ob mice was stimulated with TDM for up to 3 days. ( b ) Effect of TDM stimulation on mRNA expression of Mincle , Tnfa , fibrosis-related genes ( Tgfb1 , Pdgfb , Timp1 ) and Acta2 . Values are mean±s.e.m. The data are analysed by unpaired t -test; n =4, ** P <0.01, NS, not significant. ( c , d ) Co-culture experiments of peritoneal macrophages and adipose tissue fibroblasts. ( c ) Illustration of the co-culture experiments using peritoneal macrophages and CD45 − CD31 − cells in SVF, rich in fibroblasts, prepared from epididymal fat tissue of ob/ob mice using the magnetic cell sorting system (MACS). The cells were stimulated with TDM for up to 7 days. ( d ) Effect of TDM stimulation on mRNA expression of Acta2 and Col1a1 (collagen I). Values are mean±s.e.m. The data are analysed by unpaired t -test; n =4, ** P <0.01. Full size image Mincle-stimulated interstitial fibrosis in adipose tissue We next examined whether stimulation of Mincle is sufficient to induce interstitial fibrosis in adipose tissue in vivo . Emulsion containing TDM or vehicle was injected directly into epididymal fat tissue of Mincle KO and wild-type mice on a SD. Seven days after the injection, Masson’s trichrome staining revealed extensive interstitial fibrosis in TDM-treated wild-type mice, which was markedly suppressed in TDM-treated Mincle KO mice ( Fig. 7a,b ). By immunofluorescent staining, TDM-treated wild-type mice exhibited the CLS formation, where macrophage-surrounding adipocytes were negative for perilipin staining, which was closely associated with collagen deposition ( Fig. 7c ). Moreover, we injected the emulsion into epididymal fat tissue of COL/EGFP transgenic (Tg) mice, which express EGFP exclusively in collagen I-producing cells. We observed that a number of EGFP-positive cells were accumulated around the CLS in TDM-treated mice ( Fig. 7d ). In TDM-treated wild-type mice, Mincle and Itgax mRNA expression was markedly induced throughout the experimental period, whereas Mrc1 mRNA expression was gradually decreased ( Fig. 7e ). mRNA expression of Acta2 and collagens was gradually increased up to day 7 ( Fig. 7f ). Notably, there was no upregulation of these genes in TDM-treated Mincle KO mice ( Fig. 7f ). Collectively, these observations suggest that Mincle stimulation is capable of inducing interstitial fibrosis in adipose tissue in vivo . 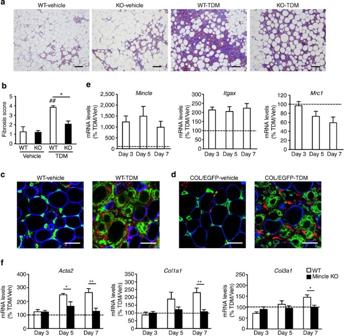Figure 7: Mincle-stimulated interstitial fibrosis in adipose tissue. Emulsion containing TDM or vehicle was injected into epididymal fat tissue ofMincleKO and wild-type mice. (a,b) Representative Masson’s trichrome staining (a) and semiquantitative analysis of interstitial fibrosis (b) of epididymal fat tissue 7 days after injection. Original magnification, × 100; Scale bar, 100 μm. Values are mean±s.e.m. The data are analysed by ANOVA followed by Tukey–Kramer test;n=4 to 5,##P<0.01 versus WT–vehicle, *P<0.05. (c) Representative immunofluorescent staining of F4/80 (green), perilipin (blue) and collagen I (red) in wild-type mice treated with TDM or vehicle. Original magnification, × 600; Scale bar, 50 μm. (d) Representative immunofluorescent staining of F4/80 (green), perilipin (blue) and EGFP (red) in COL/EGFP Tg mice treated with TDM or vehicle. Original magnification, × 600; Scale bar, 50 μm. (e,f) Time course of mRNA expression up to 7 days after injection. mRNA expression ofMincle,ItgaxandMrc1in wild-type mice (e) and that ofActa2,Col1a1andCol3a1(collagen III) inMincleKO and wild-type mice (f). Values are mean±s.e.m. The data are analysed by unpairedt-test;n=4 to 5, *P<0.05, **P<0.01. Figure 7: Mincle-stimulated interstitial fibrosis in adipose tissue. Emulsion containing TDM or vehicle was injected into epididymal fat tissue of Mincle KO and wild-type mice. ( a , b ) Representative Masson’s trichrome staining ( a ) and semiquantitative analysis of interstitial fibrosis ( b ) of epididymal fat tissue 7 days after injection. Original magnification, × 100; Scale bar, 100 μm. Values are mean±s.e.m. The data are analysed by ANOVA followed by Tukey–Kramer test; n =4 to 5, ## P <0.01 versus WT–vehicle, * P <0.05. ( c ) Representative immunofluorescent staining of F4/80 (green), perilipin (blue) and collagen I (red) in wild-type mice treated with TDM or vehicle. Original magnification, × 600; Scale bar, 50 μm. ( d ) Representative immunofluorescent staining of F4/80 (green), perilipin (blue) and EGFP (red) in COL/EGFP Tg mice treated with TDM or vehicle. Original magnification, × 600; Scale bar, 50 μm. ( e , f ) Time course of mRNA expression up to 7 days after injection. mRNA expression of Mincle , Itgax and Mrc1 in wild-type mice ( e ) and that of Acta2 , Col1a1 and Col3a1 (collagen III) in Mincle KO and wild-type mice ( f ). Values are mean±s.e.m. The data are analysed by unpaired t -test; n =4 to 5, * P <0.05, ** P <0.01. Full size image Since numerous studies have shown that obesity induces chronic inflammation in adipose tissue [1] , [2] , it is not surprising that, similar to various organs and tissues under chronic inflammation, adipose tissue exhibits interstitial fibrosis during the development of obesity. In line with this, recent evidence showed overproduction of extracellular matrix components in adipose tissue from obese animals and humans, which is implicated in systemic insulin resistance and hepatic steatosis [6] , [22] , [23] , [24] . However, little is known about how adipose tissue fibrosis is regulated in response to overnutrition. In this study, we provide evidence suggesting that Mincle is a novel regulator of adipose tissue fibrosis. Although macrophages are crucial for the regulation of tissue fibrosis, macrophages can promote and regress tissue fibrosis depending on the context [25] . Our data suggest that macrophages promote adipose tissue fibrosis through Mincle during the development of obesity. We previously reported that a paracrine loop between adipocytes and macrophages establishes a vicious cycle that augments inflammatory changes in adipose tissue during the development of obesity [5] . CLS represents a unique structure where adipocytes and macrophages crosstalk in close proximity in obese adipose tissue in vivo , thereby accelerating adipose tissue inflammation. The data of this study suggest that CLS is an important origin of fibrosis as well as inflammation in adipose tissue. This notion is supported by our recent observations that the CLS-like histological structure in the liver of nonalcoholic steatohepatitis in mice and humans, which may be involved in the fibrogenesis of the liver [26] . Given that Mincle expression is localized to macrophages constituting CLS and that residual lipid droplets of dead adipocytes are scavenged by macrophages within CLS, Mincle can sense as-yet-unidentified endogenous ligands that are released as danger signals from dead adipocytes in the interaction between adipocytes and macrophages. This is the first report to elucidate the role of Mincle, a pathogen sensor for pathogenic fungi and Mycobacterium tuberculosis , in sterile inflammation. Considering the structural and functional similarities between CLS and mycobacterial granuloma, it is interesting to compare the role of Mincle under those conditions. In this regard, our data indicate the critical role of Mincle in CLS formation in adipose tissue, which is reminiscent of the recent report by Ishikawa et al . that Mincle is essential for the TDM-induced granuloma formation in lung [13] . Moreover, CLS in adipose tissue and granuloma structure in lung are accompanied by tissue fibrosis. Taken together, it is conceivable that Mincle has a role in metabolic stress- as well as pathogen-induced sustained cell-to-cell communication within CLS, thereby contributing to tissue remodelling. It is important to know how Mincle-expressing macrophages are involved in fibrogenesis in adipose tissue. Stimulation of Mincle with TDM activates Syk in macrophages to increase expression of fibrosis-related genes as well as proinflammatory cytokines. These observations are consistent with previous studies that activation of Syk can induce TGFβ production in macrophages and dendritic cells [27] , [28] . On the other hand, Mincle is selectively expressed in proinflammatory M1 macrophages and localized to some of the macrophages constituting CLS in obese adipose tissue, whereas antiinflammatory M2 macrophages, not M1 macrophages, are considered to contribute to tissue repair and remodelling. These observations led us to speculate that Mincle-expressing macrophages could be a novel subpopulation of adipose tissue macrophages contributing to tissue remodelling under chronic inflammatory conditions. This notion is supported by recent evidence that adipose tissue macrophages exhibit mixed phenotypes of M1 and M2 in obese humans and mice [29] , [30] , [31] . Interestingly, our data show that Mincle contributes to CLS formation and fibrogenesis without affecting macrophage polarization in obesity-induced adipose tissue inflammation. Since Mincle expression is quite low in adipose tissue from healthy lean mice, it is conceivable that Mincle-expressing macrophages are involved in pathological tissue remodelling in adipose tissue. Fibrogenesis is a complex process caused by a variety of cells including myofibroblasts, immune cells and parenchymal cells. In terms of adipose tissue fibrosis, it is known that expression of collagen I and III is largely derived from SVF rather than adipocytes [32] . However, little is known about myofibroblasts in adipose tissue. In addition, myofibroblasts are derived from different cell types such as resident fibroblasts and fibrocytes, depending upon organs and tissues [20] . In this study, we observed increased number of αSMA-positive cells or myofibroblasts in obese adipose tissue. It is, therefore, interesting to know the origin of myofibroblasts in obese adipose tissue. In this regard, human preadipocytes are reported to be a source of ECM [33] , [34] , [35] . It is also important to understand the molecular mechanisms underlying myofibroblast formation during the development of obesity. Our data suggest that Mincle stimulation in macrophages effectively increases myofibroblast formation in SVF probably through the interaction between macrophages and fibroblasts. Consistently, several studies point to the role of macrophages in promoting fibroblastic phenotype and ECM production in human preadipocytes [33] , [34] , [35] . Taken together with recent observations that activation of hypoxia-inducible factor-1 in adipocytes contributes to interstitial fibrosis in adipose tissue [8] , Mincle in macrophages may link obesity-induced adipocyte damages with myofibroblast formation. Storing excessive energy as triglyceride is a fundamental function of adipose tissue. In response to nutritional conditions, lipid metabolism in adipose tissue is tightly regulated by hormones and the sympathetic nervous system. For instance, catecholamines induce adipocyte lipolysis to supply free fatty acids as fuel to other organs during the fasted state. On the other hand, insulin suppresses adipocyte lipolysis and facilitates lipogenesis in adipose tissue during the fed state [3] . In addition, accumulating evidence suggests that chronic inflammation in adipose tissue can induce ectopic lipid accumulation through several mechanisms [3] , [4] . First, obesity-induced chronic inflammation causes insulin resistance in adipose tissue [1] , [2] . Second, proinflammatory cytokines such as TNFα can directly induce lipolysis in adipocytes [5] . Finally, adipose tissue fibrosis may limit the expandability of adipose tissue during the development of obesity [6] . Divoux et al . [32] reported that adipose tissue fibrosis is negatively correlated with adipocyte diameters in human adipose tissue. It is also known that adipose tissue macrophage infiltration is associated with hepatic lipid accumulation in humans [36] . Moreover, we observed that melanocortin 4 receptor-deficient mice fed a HFD exhibit accelerated adipose tissue inflammation with interstitial fibrosis, which may contribute to excessive lipid accumulation in the liver [24] . In line with this, Mincle KO mice are protected against obesity-induced adipose tissue fibrosis and ectopic lipid accumulation in the liver. We also found that serum FFA concentrations are significantly decreased in Mincle KO mice relative to wild-type mice. All these data support the notion that increased lipid-storage capacity of adipose tissue in Mincle KO mice may cause less efflux of FFA from adipose tissue to the liver. Our data highlight the role of Mincle as a novel mechanism of how chronic inflammation induces ectopic lipid accumulation in obesity. It is important to know which organ is responsible for the ameliorated glucose tolerance in Mincle KO mice. In this study, Mincle KO mice exhibit better glucose tolerance and lower serum insulin concentrations than wild-type mice as early as 16 weeks after HFD feeding, when there is a marked reduction of hepatic steatosis in Mincle KO mice. Consistently, insulin sensitivity is significantly increased in the liver and tends to be ameliorated in adipose tissue and skeletal muscle as well as in Mincle KO mice relative to wild-type mice. These observations support the notion that activation of Mincle in adipose tissue triggers ectopic lipid accumulation and insulin resistance in the liver, thereby inducing systemic glucose intolerance. On the other hand, we do not exclude the possibility that Mincle in non-adipose tissues has a role in obesity-induced ectopic lipid accumulation and insulin resistance, since obesity also induces Mincle expression in liver to a lesser extent than adipose tissue. Further studies are required to elucidate the molecular mechanisms underlying Mincle-mediated glucose intolerance in obesity. On the basis of our observations, we hypothesize a role of Mincle in adipose tissue inflammation in obesity as follows ( Fig. 8 ). During the development of obesity, Mincle expression is induced mainly through TLR4 in infiltrated macrophages as we previously reported [18] . Activated by an endogenous ligand released from dying adipocytes, Mincle is involved in macrophage aggregation to form CLS, where there is a sustained interaction between adipocytes and macrophages. Mincle activation also induces expression of fibrosis-related genes through Syk, thereby leading to myofibroblast formation possibly through intercellular communication between macrophages and fibroblasts. As a result, overproduction of ECM may limit the HFD-induced hypertrophy of adipocytes, which has a role in lipid accumulation in the liver and glucose intolerance. 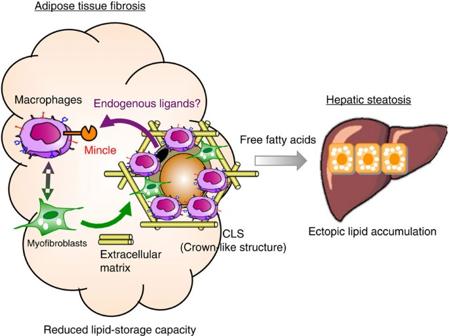Figure 8: Potential role of Mincle in obesity-induced adipose tissue inflammation. During the development of obesity, Mincle expression is induced in infiltrated macrophages and activated by an endogenous ligand released from dying adipocytes. Mincle is involved in macrophage aggregation to form CLS, and Mincle activation also induces expression of fibrosis-related genes thereby leading to myofibroblast formation. As a result, overproduction of ECM may limit the HFD-induced hypertrophy of adipocytes, which has a role in lipid accumulation in the liver and glucose intolerance. Figure 8: Potential role of Mincle in obesity-induced adipose tissue inflammation. During the development of obesity, Mincle expression is induced in infiltrated macrophages and activated by an endogenous ligand released from dying adipocytes. Mincle is involved in macrophage aggregation to form CLS, and Mincle activation also induces expression of fibrosis-related genes thereby leading to myofibroblast formation. As a result, overproduction of ECM may limit the HFD-induced hypertrophy of adipocytes, which has a role in lipid accumulation in the liver and glucose intolerance. Full size image In summary, we demonstrated in this study that Mincle has a critical role in HFD-induced CLS formation and adipose tissue fibrosis, which may reduce lipid-storage capacity in adipose tissue and enhance ectopic lipid accumulation. Our data also suggest that Mincle in macrophages would be a novel therapeutic target to prevent or treat obesity-induced adipose tissue inflammation and metabolic derangement. Reagents All reagents were purchased from Sigma-Aldrich (St Louis, MO) or Nacalai Tesque (Kyoto, Japan) unless otherwise noted. Animals The Mincle KO mice and enhanced green fluorescence protein ( Egfp ) Tg mice on the C57BL/6J genetic background were kindly provided by Drs Shizuo Akira and Masaru Okabe (Osaka University) [16] , [37] , respectively. We crossed these mice to generate the Mincle KO- Egfp Tg mice for the BMT experiments. Eight-week-old C57BL/6J- ob/ob and wild-type mice were purchased from Japan SLC (Shizuoka, Japan). They were maintained in a temperature-, humidity- and light-controlled room (12 h light/dark cycles), allowed free access to water and standard chow (CE-2; 343.1 kcal per 100 g, 12.6% energy as fat; CLEA Japan, Tokyo, Japan). Ten-week-old animals were fed either an SD (CE-2) or HFD (D12492; 556 kcal per 100 g, 60% energy as fat; Research Diets, New Brunswick, NJ) for 8, 16 and 50 weeks. The COL/EGFP Tg mice on the C57BL/6J background, which express EGFP exclusively in collagen I-producing cells, were used to detect myofibroblasts [38] . All animal experiments were approved by the Institutional Animal Care and Use Committee of Tokyo Medical and Dental University (No.2011-207C, No.0140016A). We used male 9–11-week-old mice with a C57BL/6J background in all experiments in the present study unless otherwise noted. Histological analysis The epididymal fat tissue and liver were fixed with neutral-buffered formalin and embedded in paraffin. Two-micrometre thick sections were stained with hematoxylin and eosin, Masson’s Trichrome, or Sirius red. For the measurement of adipocyte cell size, more than 200 cells were counted per each section using an image analysis software (WinRoof; Mitani, Tokyo, Japan). Fibrosis and αSMA-positive area were measured by an image analysis software (Dynamic Cell Count; Keyence, Osaka, Japan). The presence of F4/80-positive macrophages in epididymal fat tissue was detected immunohistochemically using the rat monoclonal anti-mouse F4/80 antibody kindly provided by Dr Motohiro Takeya (Kumamoto University) [39] , [40] . The number of F4/80-positive cells was counted in more than 10 mm 2 area of each section and expressed as the mean number per mm 2 . The CLS density was obtained by counting the total numbers of CLS and adipocytes in each section, which was expressed as CLS number per 10,000 adipocytes [41] . Antibodies used in this study for immunohistochemistry are listed in Supplementary Table 2 . To evaluate the TDM-induced adipose tissue fibrosis, the sections were graded semiquantitatively (scores 0 to 4) according to the Masson’s trichrome-positive area (0=none, 1=weak, 2=mild, 3=moderate, 4=severe). The representative histological images for the respective score values were shown in Supplementary Fig. 9 . The quantitative histological analysis was performed by three investigators who had no knowledge of the origin of the slides. In situ hybridization In situ hybridization for Mincle mRNA was performed as reported [42] . Paraffin-embedded tissue blocks from epididymal fat tissue were sectioned at 8 μm. The sections were fixed with 4% paraformaldehyde for 15 min, treated with 8 μg ml −1 proteinase K for 30 min at 37 °C, re-fixed with 4% paraformaldehyde and then acetylated with 0.25% acetic anhydride for 10 min. Hybridization was performed with probes at concentrations of 300 ng ml −1 at 60 °C for 16 h. After hybridization, the sections were washed in 5 × saline sodium citrate (SSC) at 60 °C for 20 min and then in 50% formamide and 2 × SSC at 60 °C for 20 min, followed by treatment with 50 μg ml −1 RNaseA for 30 min at 37 °C. After the sections were further washed several times with 2 × SSC and 0.2 × SSC, they were incubated with anti-DIG AP conjugate (Roche) for 1 h at room temperature. After washing twice, colouring reactions were performed with NBT/BCIP solution (Roche) overnight. Several sections were double stained with a macrophage marker, Iba1. Flow cytometric analyses Flow cytometric analyses of SVF were performed as described [43] , [44] . In brief, the epididymal fat tissue was collected and cut into small pieces and incubated for 20 min in collagenase solution (2 mg ml −1 of collagenase type 2 (Worthington, Lakewood, NJ)) with gentle shaking. After filtering though a 180-μm mesh, we centrifuged it and resuspended in phosphate-buffered saline (PBS). We washed the dissociated SVF twice with PBS, incubated them for 10 min in erythrocyte-lysing buffer and filtered it through a 70-μm mesh. Cells were sorted using FACSAriaII (BD Biosciences, San Jose, CA) and used for mRNA expression analysis. Mincle-expressing cells were analysed using FACSCantoII (BD Biosciences) and FlowJo 7.2.2. software (Tomy Digital Biology, Tokyo, Japan). Mincle-expressing cells were identified by anti-Mincle antibody (clone 4A9; MBL, Nagoya, Japan) labelled with Lightning-Link Atto-488 (Innova Biosciences, Cambridge, UK). Other antibodies used in flow cytometric analyses were listed in Supplementary Table 3 . Confocal microscopic analysis For confocal microscopic analysis, isolated tissue pieces were fixed in 4% formaldehyde and permeabilized with 0.5% Triton X-100. The specimens were then blocked with 1% BSA and incubated with a pair of primary antibodies and then with the respective secondary antibodies. The stainings were examined by using the FluoView FV10i confocal microscope system (Olympus, Tokyo, Japan). Collagen content in adipose tissue Total collagen content in adipose tissue was measured using a commercially available kit (The QuickZyme total collagen assay; QuickZyme Biosciences, Leiden, Netherlands). Triglyceride content in liver Total lipids in the liver were extracted using ice-cold chloroform and methanol, 2:1 (v/v). Triglyceride content in the liver content was measured using an enzymatic assay kit (Wako Pure Chemical Industries, Osaka, Japan). Glucose and insulin tolerance tests Glucose tolerance test was performed after an 18-h fast. Blood glucose concentrations were measured at 0, 15, 30, 60, 90 and 120 min after intraperitoneal injection of glucose (2 g kg −1 body weight) by a blood glucose test meter (Glutest PRO R; Sanwa-Kagaku, Nagoya, Japan). For insulin tolerance test, insulin (0.5 U kg −1 body weight of Humulin R-Insulin; Eli Lilly, Indianapolis, IN) was injected intraperitoneally after a 1-h fast. Blood glucose concentrations were measured 0, 15, 30, 60, 90 and 120 min after the injection. Western blotting of Akt Western blotting was performed as described [45] . In brief, mice with food deprivation for 16 h were injected with insulin (0.5 U kg −1 body weight of Humulin R-Insulin; Eli Lilly) or PBS via the postcaval vein. Liver, soleus muscle and epididymal fat tissue were removed 1, 2 and 3 min after the injection, respectively. Immunoblotting was performed using anti-phospho-Akt (Thr308) antibody (Cell Signaling Technology, Danvers, MA) and anti-Akt antibody (Santa Cruz Biotechnology, Santa Cruz, CA). Immunoblot images were quantified using ImageQuant LAS 4000 mini (Fujifilm, Tokyo, Japan). Representative uncropped blots are shown in Supplementary Fig. 10 . Serum analysis Serum FFA and ALT, and insulin concentrations were measured using a standard enzymatic assay or a commercially available enzyme-linked immunosorbent assay kit. TDM stimulation For stimulation of thioglycollate-elicited peritoneal macrophages or SVF from epididymal fat tissue of ob/ob mice, TDM dissolved in chloroform at 1 mg ml −1 were diluted in isopropanol and added on 12- or 48-well culture plates (5 or 1.25 μg of TDM per well, respectively), followed by evaporation of the solvent as described [13] , [46] . In some experiments, peritoneal macrophages were co-cultured with adipose tissue fibroblasts (CD45 − CD31 − cells prepared from SVF of ob/ob mice using the magnetic cell sorting system (MACS; Miltenyi Biotec, Auburn, CA)). For in vivo experiments, the emulsion containing TDM (10 μg; ref. 13 ) was directly injected into epididymal fat tissue. Three, five and seven days after the injection, the epididymal fat tissue was collected and subjected to gene expression analysis and Masson’s trichrome and immunofluorescent stainings. Quantitative real-time PCR Quantitative real-time PCR was performed as described [18] . In brief, total RNA was extracted from the tissues or cultured cells using Sepasol reagent and 10 ng of cDNA was used for real-time PCR amplification with SYBR GREEN detection protocol in a thermal cycler (StepOne Plus, Applied Biosystems, Foster City, CA). Primers used in this study are listed in Supplementary Table 4 . Data were normalized to the 36B4 levels, and analysed using the comparative CT method. Microarray analysis Microarray analysis was performed using Affymetrix GeneChip Mouse Genome 430 2.0 Arrays according to the manufacturer’s instructions. Normalization of gene expression data was processed using the Affymetrix Microarray Analysis Suite 5.0 (MAS5) algorithms. Differentially expressed genes were selected with fold change and P value (fold change >2, P <0.01). Pathway and gene ontology analyses were performed using the Reactome functional protein interaction database ( http://www.reactome.org/ ). BMT experiments BMT was performed as described [39] . In brief, bone marrow cells obtained from Mincle KO- Egfp Tg mice and Egfp Tg mice were washed three times with cold PBS and injected intravenously (1.8 × 10 6 cells) into 7.5 Gy irradiated 8-week-old male wild-type recipient mice. After 4 weeks, the substitution rate of bone marrow cells was determined by counting EGFP-positive cells in the peripheral blood and then the mice were fed a HFD for 16 weeks. Statistical analysis Data are presented as the mean±s.e.m., and P <0.05 and P <0.01 were considered statistically significant. Statistical analysis was performed using analysis of variance followed by Tukey–Kramer test. Unpaired t -test was used to compare two groups. In the GTT and ITT data, the entire curves were analysed using repeated-measures analysis of variance adjusted with degrees of freedom by Huynh and Fedlt if the Mauchly’s sphericity test is significant ( P <0.05). How to cite this article: Tanaka, M. et al . Macrophage-inducible C-type lectin underlies obesity-induced adipose tissue fibrosis. Nat. Commun. 5:4982 doi: 10.1038/ncomms5982 (2014). Accession codes: Microarray data have been deposited in the NCBI Gene Expression Omnibus (GEO) under accession code GSE52338 .